Formation of nitrogen-doped graphene nanoscrolls by adsorption of magnetic γ-Fe2O3nanoparticles Graphene nanoscrolls are Archimedean-type spirals formed by rolling single-layer graphene sheets. Their unique structure makes them conceptually interesting and understanding their formation gives important information on the manipulation and characteristics of various carbon nanostructures. Here we report a 100% efficient process to transform nitrogen-doped reduced graphene oxide sheets into homogeneous nanoscrolls by decoration with magnetic γ-Fe 2 O 3 nanoparticles. Through a large number of control experiments, magnetic characterization of the decorated nanoparticles, and ab initio calculations, we conclude that the rolling is initiated by the strong adsorption of maghemite nanoparticles at nitrogen defects in the graphene lattice and their mutual magnetic interaction. The nanoscroll formation is fully reversible and upon removal of the maghemite nanoparticles, the nanoscrolls return to open sheets. Besides supplying information on the rolling mechanism of graphene nanoscrolls, our results also provide important information on the stabilization of iron oxide nanoparticles. Graphene-based materials have emerged as a key material in nanotechnology and continuously find new areas of applications [1] , [2] , [3] , [4] , [5] . Reduced graphene oxide (rGOx) nanoscrolls are new members in the graphene family, formed by rolling single graphene sheets from one side or from a corner to form Archimedean-type spirals, more commonly known as Swiss rolls. Owing to their unique structure, graphene nanoscrolls are predicted to retain the excellent high conductance of single graphene sheets [6] . This is in contrast to single-walled carbon nanotubes where structural constraints on the electron wavefunctions make them either metallic or semiconducting, depending on their diameter and chirality [7] . Concurrent with unique electronic properties, the appropriate layer spacing of nanoscrolls might allow for energy storage applications [8] , [9] . Despite fascinating properties and a handful of theoretical studies of graphene nanoscrolls [10] , [11] , [12] , [13] , [14] , only few experimental studies [15] , [16] , [17] , [18] are reported for rGOx nanoscrolls. Viculis et al . [17] showed that exfoliation of graphite by alkali metals followed by very strong sonication led to the formation of nanoscrolls, whereas Wang et al . [18] showed that the aggregation of Ag particles on graphene sheets together with high-power sonication initiated the rolling of the rGOx nanoscrolls. However, in none of these studies a thorough explanation is given on how and why the graphene sheets form rolled structures, and with few exceptions [15] the efficiency is low. Here we describe a simple and efficient solution-based process, complemented by a detailed analysis of the rolling mechanism. We show that symmetric nitrogen-doped (13%) rGOx(N-rGOx) nanoscrolls are formed by decorating N-rGOx with magnetic iron oxide particles in the form of maghemite γ-Fe 2 O 3 . In contrast, we show that a similar decoration by less magnetic hematite (α-Fe 2 O 3 ) or non-magnetic palladium oxide particles never leads to any rolling. Similarly, control experiments with low-level or non-N-rGOx decorated by maghemite particles show no rolling, indicating that the nitrogen defects are largely involved in the rolling mechanism. Different to earlier reports [18] and to theoretical predictions [14] , we show that the rolling process is fully reversible and that the N-rGOx can be fully transformed back to open graphene sheets by the removal of iron oxide particles through acid washing. We conclude that the rolling is initiated by the strong adsorption of maghemite nanoparticles at nitrogen defects in the graphene lattice and their mutual magnetic interaction. Our experimental observations are supported by ab initio density functional theory calculations. Physical properties of the nanoscrolls The basis of our study relies on attempts to decorate N-rGOx sheets by hematite and tungsten oxide nanoparticles to obtain materials appropriate for water oxidation. In the context of this work, we have come across a very peculiar effect. When the N-rGOx sheets unintentionally were decorated by maghemite nanoparticles, a metastable form of hematite that stabilizes under slightly different conditions, the micrographs of transmission electron microscopy (TEM) consistently revealed the presence of almost 100% of N-rGOx nanoscrolls instead of the commonly open N-rGOx sheets obtained by hematite decoration. Both hematite and maghemite have technologically interesting properties: hematite is used as catalyst for water oxidation [19] , [20] or as paint pigment, whereas maghemite is used as a contrast media in magnetic resonance or as magnetic recording media [21] . Despite many similarities, the two materials also display significant differences. Hematite crystallizes in a rhombohedral structure, whereas maghemite forms a cubic structure [21] , [22] . The difference in crystal structure rationalizes the magnetic properties of maghemite and hematite, where maghemite is ferrimagnetic and displays a much stronger magnetic moment (~540 mT) than the weakly ferromagnetic hematite (~1 mT). However, nanoparticles of both maghemite and hematite exhibit superparamagnetic behaviour, as each nanoparticle forms single magnetic domains [23] , [24] . We show in our study that the magnetically interacting maghemite particles and their strong adsorption on the N-rGOx sheets seem to be the main reasons for the formation of the N-rGOx nanoscrolls. The rolling mechanism of N-rGOx nanoscrolls is revealed by conducting a large number of control experiments to tune and test the synthesis conditions. The conditions leading to the highest ratio of, and most symmetric, nanoscrolls were achieved by adding iron(III) chloride, tungsten hexacarbonyl, and polyvinylpyrrolidone (PVP) and hydrazine into a N-rGOx methanol dispersion, followed by heating under reflux for 24 h (see Methods ). The scheme for the optimal conditions leading to nearly 100% (the only exception was some few very large graphene sheets, >5 μm) of N-rGOx nanoscrolls is shown in Fig. 1 (route a), together with the conditions used when hematite is formed and the decorated N-rGOx remain as open flat sheets ( Fig. 1 , route b). The formation of maghemite and hematite can be controlled by slight changes in the solution. When using a pure methanol solution, formation of maghemite particles is observed, whereas replacing a part of the methanol by water leads to the formation of hematite. 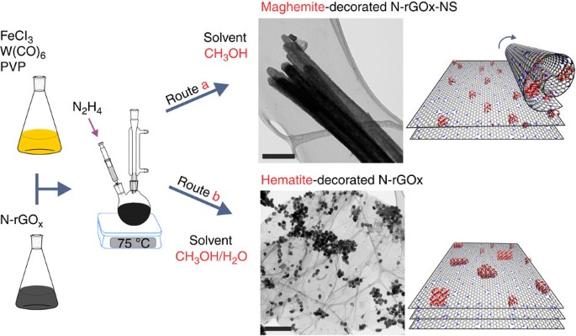Figure 1: Schematic process for the adsorption of iron oxide nanoparticles. (route a) Maghemite-decorated nitrogen doped reduced graphene oxide (N-rGOx) nanoscrolls, and (route b) hematite-decorated N-rGOx sheets. Figure 1: Schematic process for the adsorption of iron oxide nanoparticles. (route a) Maghemite-decorated nitrogen doped reduced graphene oxide (N-rGOx) nanoscrolls, and (route b) hematite-decorated N-rGOx sheets. Full size image The TEM micrograph in Fig. 1 (route a) shows N-rGOx nanoscrolls with diameters of about 38 nm decorated by small maghemite nanoparticles, in the range of 3–5 nm, whereas the hematite nanoparticles on the N-rGOx sheets are larger and are in the range of 25–40 nm ( Fig. 1 , route b). The nanoscrolls tend to arrange in bundles with up to 20 scrolls in each bundle ( Supplementary Figs S1–S3 ). Statistical analysis of >100 nanoscrolls reveals an average diameter of ~38±1 nm (s.d., σ =10.5 nm; see histogram in Supplementary Fig. S3a ). The X-ray diffraction patterns of N-rGOx nanoscrolls and N-rGOx sheets ( Fig. 2a ) show diffraction patterns characteristic for maghemite and hematite crystallized in cubic and rhombohedral structures, respectively [22] . From Scherrer’s formula [25] , we estimate the diameter of the nanoparticles to be 3.5 nm for the maghemite particles and 25 nm for the hematite particles, in good agreement with the TEM micrographs. By simply calculating the number of spirals (turns) of a single nanoscrolls, considering the average diameter of 38 nm, and assuming an interlayer distance of 5 nm (considering the particle size, C-Fe length and 0.3 Å as van der Waals interaction with the next graphene layer), the resulting nanoscrolls may consist of a single graphene sheets rolled ~3–5 turns. This estimation seems to be consistent with TEM micrographs in which the maghemite-decorated N-rGOx nanoscrolls are seen as transparent material under electron irradiation. Further support for the fact that the structures are indeed formed as nanoscrolls is obtained using scanning transmission electron microscopy and high resolution TEM (HRTEM) using diffraction, thickness and carbon contrast for the HRTEM mode ( Supplementary Fig. S4 ) and the corresponding simulations of the HRTEM data ( Supplementary Fig. S5 ). In Supplementary Fig. S4d , the stacked carbon atoms in the graphene planes parallel to the electron beam are consistent with the Archimedean structures simulated in Supplementary Fig. S5 (see Supplementary Note 1 ). 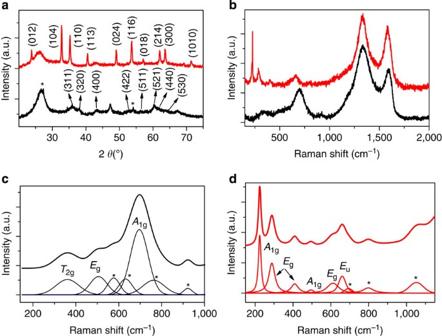Figure 2: X-ray and Raman characterization. (a) X-ray diffraction pattern of maghemite-decorated rolled N-rGOx nanoscrolls (red line) and hematite-decorated N-rGOx sheets (black curve). (b) Observed Raman spectrum of decorated N-rGOx. Peak-fitted and assigned spectrum of (c) maghemite-decorated rolled N-rGOx nanoscrolls and (d) hematite-decorated N-rGOx, (peaks originating from W-O vibrational modes are assigned with ‘*’). Figure 2: X-ray and Raman characterization. ( a ) X-ray diffraction pattern of maghemite-decorated rolled N-rGOx nanoscrolls (red line) and hematite-decorated N-rGOx sheets (black curve). ( b ) Observed Raman spectrum of decorated N-rGOx. Peak-fitted and assigned spectrum of ( c ) maghemite-decorated rolled N-rGOx nanoscrolls and ( d ) hematite-decorated N-rGOx, (peaks originating from W-O vibrational modes are assigned with ‘*’). Full size image The formation of maghemite and hematite in the two morphologically different samples is further supported by the Raman spectra of maghemite-decorated N-rGOx nanoscrolls and hematite-decorated N-rGOx sheets shown in Fig. 2b–d , respectively. The high wave number region in Raman spectra of both samples ( Fig. 2b ) comprises a D-band and a G-band region and can be fitted by a 4-peak model with peaks at 1,185, 1,339, 1,470 and 1,584 cm −1 in agreement with previous reports of nitrogen-doped carbon nanostructures [26] , [27] . More importantly, the low-frequency region of maghemite-decorated N-rGOx nanoscrolls in Fig. 2c displays features that match well with the Raman active modes of maghemite ( A 1g + E g +3 T 2g ) with the most pronounced mode, A 1g , at ~696 cm −1 . Two weaker peaks at ~506 and ~361 cm −1 are assigned to the T 2g and E g modes [28] , respectively, but are slightly down-shifted owing to the interaction of nanoparticles with graphene. The low-frequency region of hematite-decorated N-rGOx sheets in Fig. 2d displays characteristic features of hematite [29] , [30] , [31] , with the largest peaks at 224 and 289 cm −1 . Fig. 2c, d display the symmetry assignment of each peak, but for a detailed analysis of the Raman spectra and a corresponding table with wavenumbers and symmetries we refer to Supplementary Table S1 . Weak peaks in the range between 400 and 1,000 cm −1 present in the Raman spectra of both types of samples are assigned to W-O vibrations [32] . According to the thermo gravimetric analysis (TGA), the loading of maghemite and hematite is around 40 mass percent for both maghemite-decorated N-rGOx nanoscrolls and hematite-decorated N-rGOx sheets, respectively ( Supplementary Fig. S7 ). The heat-induced oxidation of the rGOx around 450 °C is much more distinct and correlated to a sharper heat flow curve for the hematite-decorated N-rGOx sheets compared with the corresponding oxidation of maghemite-decorated N-rGOx nanoscrolls. This is rationalized by the fact that the sheets are much more reactive than the nanoscrolls because of their larger surface area exposed to oxygen. Mechanism of nanoscroll formation The strong magnetic moment of maghemite compared with hematite is a plausible reason for the formation of the nanoscrolls. However, we also note that the adsorbed hematite particles are significantly larger than the maghemite particles. The separation distance, and hence the size of the absorbed nanoparticles, is a key factor in the van der Waals exchange force between colloidal particles [33] . The larger size of the hematite particles might be related to a swelling mechanism of the physisorbed surfactant correlated to the introduction of water in the synthesis of the hematite particles, as described by Chen et al . [34] , [35] The swelling leads to a partial removal of the surfactant leading to the aggregation of partially unprotected hematite particles. Supplementary Fig. S8 shows the aggregation of small hematite particles into larger clusters. By changing the pH value for the synthesis, we have successfully decreased the size of the hematite particles to almost the same size as the maghemite particles (4–8 nm for hematite particles versus 3–5 nm for maghemite particles), without finding any rolled hematite-decorated N-rGOx sheets. Further support that the size does not has a decisive role for the rolling of the N-rGOx is achieved by homogeneously decorating N-rGOx sheets with palladium oxide nanoparticles having the same diameter as the maghemite particles (3–5 nm). Also, in this case no rolling is found ( Supplementary Fig. S9 ). This strengthens our hypothesis that the magnetic character of maghemite has a significant role in the rolling mechanism. The magnetic character of the maghemite-decorated N-rGOx nanoscrolls (particle size 3–5 nm) and the hematite-decorated N-rGOx sheets (particle size 4–8 nm) was probed by superconducting quantum interference device magnetization experiments. 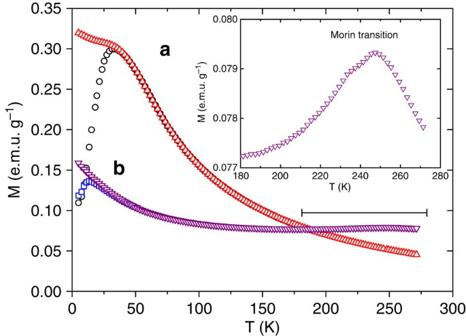Figure 3: Magnetic superconducting quantum interference device (SQUID) characterization. Magnetization versus temperature atH=1,000 Oe of (a) maghemite-decorated rolled N-rGOx nanoscrolls at ZFC conditions (black open circles) and at FC conditions (red up-triangles), and (b) hematite-decorated N-rGOx sheets at ZFC conditions (blue open squares) and at FC conditions (purple down-triangles). Inset shows an enlargement of the high temperature region for hematite-decorated N-rGOx sheets. Figure 3 , shows M versus T at zero field-cooled (ZFC) and field-cooled (FC) conditions. From these data we observe, besides the significantly stronger magnetization of the maghemite nanoparticles, that both samples show a characteristic superparamagnetic behaviour with a maximum in the ZFC curves corresponding to the blocking temperature, T B . The superparamagnetic blocking temperature is defined as the temperature at which the superparamagnetic relaxation time equals the timescale of the experimental technique [23] . The higher T B of the maghemite particles is rationalized by higher interaction between nanoparticles as well as their smaller average size compared with the hematite particles [36] . The stronger interaction between maghemite particles is further confirmed by the FC curve that flattens out at temperatures lower than T B but continue to increase for hematite nanoparticles. The plateau-shaped character for the maghemite nanoparticles is related to a transition to an ordered collective spin-glass-like state caused by the stronger dipole interactions of maghemite nanoparticles. The inset in Fig. 3 shows that hematite nanoparticles undergo a weakly pronounced Morin transition as expected for small hematite nanoparticles (see also Supplementary Fig. S10 and Supplementary Note 2 ). Figure 3: Magnetic superconducting quantum interference device (SQUID) characterization. Magnetization versus temperature at H =1,000 Oe of ( a ) maghemite-decorated rolled N-rGOx nanoscrolls at ZFC conditions (black open circles) and at FC conditions (red up-triangles), and ( b ) hematite-decorated N-rGOx sheets at ZFC conditions (blue open squares) and at FC conditions (purple down-triangles). Inset shows an enlargement of the high temperature region for hematite-decorated N-rGOx sheets. Full size image The rolling is significantly improved by adding tungsten hexacarbonyl together with the FeCl 3 salt, as displayed in Fig. 1 . A typical TEM micrograph of maghemite-decorated N-rGOx nanoscrolls without adding tungsten hexacarbonyl is shown in Supplementary Fig. S11 . Although a major fraction of the N-rGOx still is rolled, the obtained nanoscrolls are less homogeneous and have larger diameter. The complete role of tungsten is not clear, but it is known that tungsten can shift the isoelectric point of iron oxide particles to higher pH, indicating that, at the experimental conditions (pH=7.5–9), tungsten will make the iron oxide particles slightly positively charged and hence increase their interaction with the negatively charged nitrogen-doped graphene sheets. However, we note that adding only tungsten hexacarbonyl to the synthesis (without using FeCl 3 ) resulted in only tungsten-decorated N-rGOx without any signs of rolling ( Supplementary Fig. S12 ). As in the case of tungsten, the addition of PVP is not crucial for the rolling process, and by removing the PVP from route a (see Fig. 1 ) less homogeneous and larger nanoscrolls are obtained. A statistical analysis of 85 nanoscrolls in the absence of PVP reveals an average diameter of ~260±8 nm ( σ =76 nm, see histogram Supplementary Fig. S6 ). The promoting properties of PVP probably originate from its ability to attach onto the N-rGOx, thereby improving the dispersability of N-rGOx in polar environments, such as methanol or methanol–water systems. Moreover, PVP might manipulate the nucleation, growth and agglomeration of metal oxide nanoparticles by interacting with the metal oxide precursor via its hydrophilic head groups [37] , thereby preventing agglomeration of formed particles. The early steps of the nanoscroll formation, as probed by a time series analysis, are displayed in Fig. 4 , which shows TEM micrographs for synthesis that were (a) quenched in an ice bath only 1 min after the addition of hydrazine, (b) refluxed for 5 h and (c) for 24 h. We conclude that the rolling process starts by the decoration of the upper layer, which starts to roll after achieving a sufficient loading, thereby exposing the underneath layer for decoration leading to a subsequent rolling. 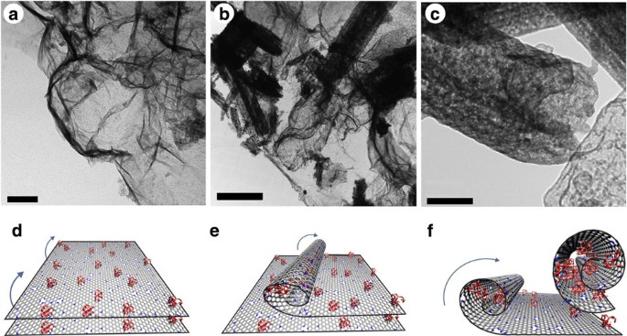Figure 4: Time sequence analysis of scroll formation. TEM micrographs showing the rolling process at different time steps for N-rGOx nanoscrolls, where edges, topological defects and doping sites act as nucleation points for iron oxide nanoparticles (a) quenched in an ice bath only 1 min after the addition of hydrazine, (b) refluxed for 5 h after the addition of hydrazine and (c) refluxed for 24 h. (d–f) Schematic illustrations for the various steps. When an optimum nanoparticles loading is reached, the net attractive forces start to roll and fold the graphene layers into cylindrical structures. Scale bars, 100, 500 and 100 nm ina,bandc, respectively. Figure 4: Time sequence analysis of scroll formation. TEM micrographs showing the rolling process at different time steps for N-rGOx nanoscrolls, where edges, topological defects and doping sites act as nucleation points for iron oxide nanoparticles ( a ) quenched in an ice bath only 1 min after the addition of hydrazine, ( b ) refluxed for 5 h after the addition of hydrazine and ( c ) refluxed for 24 h. ( d – f ) Schematic illustrations for the various steps. When an optimum nanoparticles loading is reached, the net attractive forces start to roll and fold the graphene layers into cylindrical structures. Scale bars, 100, 500 and 100 nm in a , b and c , respectively. Full size image From the results above, it seems as a high degree of maghemite decoration is important to initiate the formation of nanoscrolls. Nitrogen defects in carbon nanostructures may cause additional binding sites for metal particles [38] . In our case, the surface iron atoms in iron oxide act as Lewis acids and can readily coordinate with molecules/atoms that donate lone-pair electrons [39] . Most amines (organic compounds or functional groups that contain a basic nitrogen) are Lewis bases, such as pyrrole (C 4 H 4 NH), aniline (C 6 H 5 NH 2 ) or pyridine (C 5 H 5 N), and because of the high nitrogen incorporation (13 at%) in our samples we expect that the N-rGOx surfaces contain a large number of sites with Lewis base behaviour, which might promote the nucleation of the iron oxide nanoparticles. The role of specific nitrogen defects was elucidated by ab initio calculations to study the adsorption of iron oxide clusters on nitrogen-doped graphene sheets (N-doped GNS). Seven different nitrogen defects were introduced in the centre of the 2D graphene sheet followed by the allocation of an iron oxide (Fe 20 O 32 ) cluster near the defect ( Supplementary Figs S13 and S14 ). After geometrical relaxation the adsorption energy ( E ads ) is calculated. The results are shown in Fig. 5a , where a negative E ads signifies an energetically stable configuration. 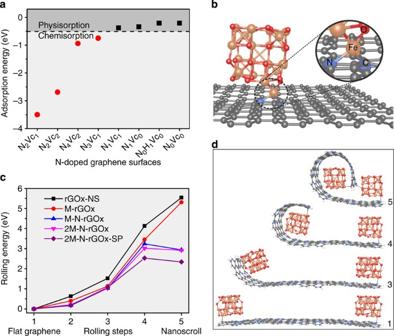Figure 5: Density functional theory (DFT) studies of scroll formation and adsorption energies. (a) Adsorption energy of an iron oxide cluster (52 atoms, Fe20O32with maghemite structure) on pristine (N0Vc0) and seven different nitrogen functionalities at a nitrogen-doped reduced graphene oxide (N-rGOx) sheet. The different functionalities refer to substitutional nitrogen atom N1Vc0, pyrrolic N1H1Vc1, pyridinic N1Vc1, triple pyridinic N3Vc1, double pyrrolic N2Vc2, pyrrolic-pyridinic N2Vc1and tetra pyridinic N4Vc2, where N (H) refers to the number of nitrogen (hydrogen) atoms and Vc the number of vacancies generated in the structure. (b) Final geometrical configuration of the N2Vc1–Fe20O32super cell. As seen, the C atoms surrounding the defect are also responsible for the favourable cluster adsorption. (c) Rolling energy of graphene nanoribbons into nanoscrolls of pure carbon-rGOx (rGOx-NS, black line), maghemite (Fe20O32)-decorated rGOx nanoscrolls (M-rGOx Red line), maghemite N-rGOx nanoscrolls (M-N-rGOx Blue line), maghemite N-rGOx nanoscrolls decorated with two Fe20O32nanoparticles, one at each end of the graphene nanoribbon (2-M-N-rGOx magenta line) and maghemite N-rGOx nanoscrolls decorated with two Fe20O32nanoparticles taking into account the spin–spin interactions of the two nanoparticles (2-M-N-rGOx-SP purple line). (d) Final geometrical structure at each rolling step of maghemite N-rGOx nanoscrolls decorated with two nanoparticles (2-M-N-rGOx). As displayed inc, the energy needed for the initial rolling decreased from 0.63 eV to 0.08 eV (in step 2) after nitrogen doping and decoration by two Fe20O32clusters the original carbon-rGOx nanoscroll. In the subsequent step 3, the rolling energy of 2-M-N-rGOx is 1.49 eV lower than that of rGOx, and the rolling energy of the full nanoscrolls structure is lowered by >3.3 eV compared with that of rGOx nanoscroll. Figure 5: Density functional theory (DFT) studies of scroll formation and adsorption energies. ( a ) Adsorption energy of an iron oxide cluster (52 atoms, Fe 20 O 32 with maghemite structure) on pristine (N 0 Vc 0 ) and seven different nitrogen functionalities at a nitrogen-doped reduced graphene oxide (N-rGOx) sheet. The different functionalities refer to substitutional nitrogen atom N 1 Vc 0 , pyrrolic N 1 H 1 Vc 1 , pyridinic N 1 Vc 1 , triple pyridinic N 3 Vc 1 , double pyrrolic N 2 Vc 2 , pyrrolic-pyridinic N 2 Vc 1 and tetra pyridinic N 4 Vc 2 , where N (H) refers to the number of nitrogen (hydrogen) atoms and Vc the number of vacancies generated in the structure. ( b ) Final geometrical configuration of the N 2 Vc 1 –Fe 20 O 32 super cell. As seen, the C atoms surrounding the defect are also responsible for the favourable cluster adsorption. ( c ) Rolling energy of graphene nanoribbons into nanoscrolls of pure carbon-rGOx (rGOx-NS, black line), maghemite (Fe 20 O 32 )-decorated rGOx nanoscrolls (M-rGOx Red line), maghemite N-rGOx nanoscrolls (M-N-rGOx Blue line), maghemite N-rGOx nanoscrolls decorated with two Fe 20 O 32 nanoparticles, one at each end of the graphene nanoribbon (2-M-N-rGOx magenta line) and maghemite N-rGOx nanoscrolls decorated with two Fe 20 O 32 nanoparticles taking into account the spin–spin interactions of the two nanoparticles (2-M-N-rGOx-SP purple line). ( d ) Final geometrical structure at each rolling step of maghemite N-rGOx nanoscrolls decorated with two nanoparticles (2-M-N-rGOx). As displayed in c , the energy needed for the initial rolling decreased from 0.63 eV to 0.08 eV (in step 2) after nitrogen doping and decoration by two Fe 20 O 32 clusters the original carbon-rGOx nanoscroll. In the subsequent step 3, the rolling energy of 2-M-N-rGOx is 1.49 eV lower than that of rGOx, and the rolling energy of the full nanoscrolls structure is lowered by >3.3 eV compared with that of rGOx nanoscroll. Full size image Among the studied defects, four different nitrogen-doping configurations, N 2 Vc 1 , N 3 Vc 1 , N 2 Vc 2 and N 4 V 2 , strongly interact with the iron oxide cluster. All these pyridinic defects exhibit the largest adsorption energies for the Fe 20 O 32 maghemite nanoparticle, and also are the most abundant in our maghemite-decorated N-rGOx nanoscrolls sample according to the X-ray photoemission spectroscopy data ( Supplementary Fig. S16 ). These results are in good agreement with our experimental observations, where high N-concentration is needed for an optimal loading of nanoparticles. Fig. 5b depicts the final geometry of the N 2 Vc 1 –Fe 20 O 32 , where the C atoms surrounding the nitrogen defect are also involved in chemical bonds between metal oxide and graphene surface ( Supplementary Fig. S14 ). This originates from the fact that the nitrogen atoms modify the local electron properties of the nearest carbon atoms [40] , [41] . Other studies point towards an asymmetric spin density caused by the introduction of nitrogen atoms [42] . Both models, however, lead to an increased chemical reactivity. As observed from Fig. 5a , the pure carbon (N 0 Vc 0 ) graphene surface system exhibits the lowest E ads, suggesting a poor interaction (a physisorption state). This is related to the homogeneous electron density along the graphene surface, contrary to the N-defects studied here, which exhibits highly localized states around the doping site. For the case when N 1 Vc 0 , N 1 H 1 Vc 1 and N 1 Vc 1 are present, steric repulsions generate low interaction between systems, suggesting that the space left by the vacancy is also needed to improve the interaction between nanoparticles and graphene. Our theoretical findings are probed by replacing the highly N-rGOx (13%) by a non-N-rGOx (GOx was treated and reduced at 750 °C in argon environment). Identical treatment conditions and procedure to decorate this sample as described in Fig. 1 (route A) led to a significantly lower maghemite loading, with only weak signs of rolling ( Supplementary Fig. S17 ). This is well in line with our theoretical calculations that the nitrogen defects promote the formation of metal nanoparticles, which in turn initiates the formation of the nanoscrolls. Besides the nitrogen defects at the N-rGOx sheets serving as initial nucleation sites for the iron oxide particles, they are involved in two additional important mechanisms; in mechanism (i), the maghemite particle can take part in a multiple binding process, indicating that after the rolling process has initiated, the unbound upper part of the maghemite particle can form additional bonds to the N-rGOx sheet. The process is visualized in Fig. 5c that displays the rolling energy of four different hydrogen-passivated nine-armchair graphene nanoribbons (9-aGNR) initially rolled as an Archimedean spiral. The first studied structure is rGOx nanoscroll, an undoped system 9-aGNR. The second one is M-rGOx, an undoped 9-aGNR decorated with iron oxide (Fe 20 O 32 ). The third one is M-N-rGOx, a nitrogen-doped 9-aGNR with pyridinic defects (N 3 Vc 1 , 14%At of N) and one Fe 20 O 32 collocated at the edge. Finally, the fourth structure is 2M-N-rGOx, the same N-doped 9-aGNR as in structure (3) but with two Fe 20 O 32 clusters at each edge of the nanoribbons. The optimized geometries are depicted in Supplementary Fig. S15 . Fig. 5c shows that the progress of rolling energy for the pure carbon graphene sheet (rGOx-NS, black line) is not linear and initially increases, but as soon as the graphene layers start to interact, the rolling energy decreases because of the mutual interlayer interaction. This trend is in agreement with a study by Braga et al . [14] More interestingly, when nitrogen defects are incorporated in the graphene lattice, and a maghemite, Fe 20 O 32 cluster, is adsorbed on the upper layer, both the energy barrier for the initial rolling step as well as the formation energy for the complete roll decreases (M-N-rGOx, blue curve). The adsorption of an additional Fe 20 O 32 cluster at the other end of the nanoribbon (2-M-N-rGOx, Fig. 5d ) lowers the formation energy further, supporting our experimental observations that a high loading seems essential for an efficient rolling. In addition, by introducing also magnetic spin–spin interaction for two neighbouring maghemite nanoparticles with opposite spins (consistent with the observed superparamagnetism for our system), we see a further decrease in the rolling energy, especially for the later steps of the rolling energy when the spin–spin interactions become larger because of the decreased distance between the maghemite nanoparticles. In mechanism (ii), we observed that the N-rGOx sheets not only promote the formation of the maghemite nanoparticles, but actually are essential for their stabilization. Hematite is the most stable phase of iron oxide, whereas maghemite is metastable and readily transforms to hematite. In nature, both hematite and maghemite can be found in minerals as well as in nanoparticle form, but it is generally accepted that a nanoparticle size-dependent transition from maghemite to hematite occurs around 10 nm [43] . Furthermore, the stabilization of maghemite nanoparticles has been observed at maghemite silica-based supports [44] . We believe that the N-rGOx sheets in our study have a similar role in stabilizing the maghemite nanoparticles by providing sufficient and suitable adsorption sites, thus inhibiting their transformation to hematite particles. This is clearly demonstrated by removing N-rGOx from the synthesis process displayed in Fig. 1 . Keeping the conditions identical otherwise leads to a formation of hematite for the methanol/water route b, whereas the methanol route a gives no formation of maghemite particles. At this condition, the absence of the N-rGOx has the consequence that the iron chloride salt simply remains dissolved in the solution after adding hydrazine and the nanoparticle formation is fully inhibited. The nanoparticle formation and their stabilization on the N-rGOx sheets is a rather complex process. The full description will be described elsewhere but we point out some important aspects; during the synthesis, the pH for both routes displayed in Fig. 1 starts around 8.5 (we realize however that the pH in pure methanol is poorly defined). With time, the pH of route a gradually increases to about 9, whereas the pH of route B lowers to about 7.5. Previous studies have shown that hydroxylation of ferric ions in solution with pH>3 leads to the formation of the thermodynamically unstable ferrihydrite [45] . Depending on the acidity of the medium, ferrihydrite transforms to different forms of iron oxide. Ferrihydrite transforms to hematite at 5≤pH≤8 [46] , with an increase in hematite particle size by an increasing acidity of the medium [47] . pH values>8.5 are expected to promote the formation of maghemite. The role of the pH is demonstrated by adding 4 μl of HCl for route A. The slight modification of the pH has the consequence that maghemite formation is interchanged by a hematite, again, with no signs of nanoscrolls formation. We note so far that the strong dipole moment of maghemite nanoparticles and their strong interaction with the nitrogen functionalities on the N-rGOx seems to be the two most important causes to initiate the formation of the nanoscrolls. Clearly, the maghemite formation requires the support of nitrogen defects on the graphene sheets and the solution pH has a significant role in directing the iron oxide crystallization towards maghemite instead of hematite. However, it is likely that water, besides balancing the pH to more neutral condition, also could have other roles in the ordering of the hematite nanoparticles by, for example, altering the molecular arrangement of methanol [48] . This could affect the polarity and size of methanol/water clusters, which are important for the solvation forces between a colloidal particle and the solvent [49] , and therefore also vital in the nanoparticle formation/aggregation. We conclude our study with a surprising observation. Earlier reports for graphene nanoscrolls indicated that the scrolls, when formed, are very stable and do not unroll or unfold, even by strong ultrasonication. As our study indicates that the adsorption of the maghemite particles is essential for the formation of the nanoscrolls, we investigated this by washing the maghemite-decorated N-rGOx nanoscrolls with acid (1:3 volume ratio of HCl: HNO 3 mixture for 24 h at 45 °C). Amazingly and in accordance with our model, the nanoscrolls go back completely to the initial open N-rGOx structure upon removal of the maghemite nanoparticles. Supplementary Fig. S18a shows the TEM micrograph of the acid-washed sample, where the quadratic particles are attributed to tungsten sheets not removed by the acid treatment ( Supplementary Figs S19 and S20 ). Acid treatment of maghemite-decorated N-rGOx nanoscrolls that do not contain tungsten shows a very nice sample comprising single or few layers of N-rGOx ( Supplementary Fig. S18b ). If the washing procedure is shortened, half-open structures can also be found, as seen in Supplementary Fig. S18c . Interestingly, we also observe that the washed samples, now comprising N-rGOx, again can be decorated with maghemite particles leading to similar formation of maghemite-decorated N-rGOx nanoscrolls as before, however, with larger diameter, probably originating from the defects introduced in the acid treatment ( Supplementary Fig. S21 ). In summary, N-rGOx nanoscrolls can form by adsorption of maghemite nanoparticles in a simple reflux method. We explain the efficient rolling process by a combination of the magnetic interaction between the maghemite nanoparticles and a strong interaction of maghemite nanoparticles with nitrogen functionalities at the graphene sheets. The rolling process is fully reversible. Upon removal of the adsorbed maghemite nanoparticles by acid treatment, the nanoscrolls return back to their original flat open structure. Our study gives important insight for the manipulation and synthesis of graphene nanoscrolls and the stabilization of iron oxide nanoparticles, which is relevant also for other geochemical, ecological and environmental processes in nature [50] . Synthesis N-rGOx was produced by a method similar to the previous reports [51] , by first producing graphene oxide (GOx), with a modified Hummers’ method. GOx was dispersed in mili-Q water (0.5 g l −1 ) by ultrasonication. Then, melamine (C 3 H 6 N 6 , 99%, Sigma-Aldrich) was added to the GOx suspension (2.5 g l −1 ) and stirred until significant agglomeration was observed. The resulting dispersion was dried at 80 °C in an oven and finally the solid material was grinded into fine powders using a mortar. The GOx–melamine complex was pyrolysed at 750 °C for 45 min under an Ar atmosphere to obtain N-rGOx. GOx was treated and reduced at high temperature (750 °C) under argon environment for 45 min. Decoration of N-rGOx by route a The N-rGOx powder was mixed with high purity methanol (1 g l −1 ) and dispersed by ultrasonication for 30 min, and was labelled as (1). Meanwhile, 77.7 μM iron(III) chloride hexahydrate (FeCl 3 , Sigma-Aldrich),60 μM tungsten hexacarbonyl(W (CO) 6 , 97%, Sigma-Aldrich) and PVP (average Mw 40,000, Sigma-Aldrich) were added in a separated flask containing methanol, stirred until dissolved completely, and were labelled as (2). Finally, both (1) and (2) were mixed under magnetic stirring, followed by a gradual heating up to 75 °C under reflux condition. When the desired temperature was reached, 0.1 ml of hydrazine (N 2 H 4 , Merck) was added to the mixture drop wise to promote the hydrolysis of FeCl 3 . The reaction was continued for a predefined time. The resulting material was washed and centrifuged in water and ethanol for several times and finally dried at 85 °C and stored for further characterization. Decoration of N-rGOx by route b The same procedure as the route A was followed but the solvent was replaced by methanol/mili-Q water mixture (1:1). PdO decoration N-rGOx was mixed with methanol (0.2 g l −1 ) and dispersed by ultrasonication for 10 min. Then, Pd acetate (1 g l −1 ) was added and sonicated again. The sonicated suspension was stirred overnight at 400 r.p.m. Tungsten decoration of N-rGOx was synthesized following route A, but FeCl 3 was completely absent in the process. Non-PVP-assisted hematite and maghemite decoration of N-rGOx was synthesized following route A and route B but in the absence of PVP. Computational methods Electronic calculations were performed using density functional theory [52] , [53] , using the generalized gradient approximation with Perdew–Burke–Ernzerhof parameterization as an exchange–correlation functional [54] , as implemented in the SIESTA code [55] . For all systems, the valence electrons were represented by a linear combination of pseudo-atomic numerical orbitals [56] using a double-ζ (DZ) basis for H, C and N atoms, and DZ-polarized basis for O and Fe atoms. In the case of iron, we have used eight valence electrons (Fe:3d74s1), and this electronic configuration has been shown to improve the description of iron oxide systems [57] . The real-space grid used for charge and potential integration is equivalent to a plane wave cut-off energy of 200 Ry, and for spin-polarized systems 350 Ry was used. Periodic boundary conditions were used and a minimum of 20 Å of vacuum was employed to avoid lateral interactions. Sampling of the 2D Brillouin zone was carried out with (1 × 3 × 3) Monkhorst–Pack grids. All structures were relaxed by conjugate gradient minimization until the maximum force was <0.05 eV Å −1 . We performed two different simulations that helped us to understand the experimental observations; these are described below. Cluster adsorption Two-dimensional (2D) periodic structures of N-doped GNS were constructed using a square super cell of 240 atoms, where seven different nitrogen-doping defects were introduced in the centre of the graphene surface: (1) substitutional nitrogen atom, N 1 Vc 0 , (2) pyrrolic, N 1 H 1 Vc 1 , (3) pyridinic, N 1 Vc 1 , (4) pyrrolic-pyridinic, N 2 Vc 1 , (5) triple pyridinic, N 3 Vc 1 , (6) double pyrrolic defect, N 2 Vc 2 and (7) tetra pyridinic, N 4 Vc 2 , where N (H) refers to the number of nitrogen (hydrogen) atoms and Vc number of vacancies generated in the structure; also the (8) undoped case is studied for comparison. The graphene super cell and N-doped defects are shown in Supplementary Fig. S13 . Previously, an iron oxide cluster containing 52 atoms (Fe 20 O 32 ) was obtained directly from iron oxide with maghemite structure, and then was geometrically optimized (The maghemite cubic cell has 56 atoms in total, where we have eliminated four Fe atoms to avoid highly uncoordinated atoms, resulting in 52 atoms (Fe 20 O 32 ) iron oxide cluster). The cluster adsorption was performed by setting the Fe 20 O 32 cluster above the seven defective sites followed by an energy minimization. Finally, we calculated the adsorption energy E ads , defined as E ads = E cmplx −( E surf + E np ), where E cmplx is the total energy of the N-doped GNS and the iron oxide cluster; the E surf ( E np ) is the total energy of the isolated N-doped GNS (iron oxide cluster). The resulting structures are depicted in Supplementary Fig. S14 . Graphene nanoscrolls Hydrogen-passivated 9-aGNRs containing 272 atoms (12 unit cells) were used as starting material. The 9-aGNRs was initially rolled as an Archimedes’ spiral, which in polar coordinates ( r,θ ) is described by the equation r=a+bθ , where a is the inner core radius, r is the radial distance, θ is the polar angle and b is the interlayer distance equal to 3.34 Å. The rolling procedure was divided in five steps until we reached a full graphene scroll, and then the structures were geometrically relaxed. To study the effect of nitrogen doping and iron oxide decoration on the rolling mechanism of graphene, we selected the following systems. ( 1 ) Structure rGOx-NS , undoped (pure carbon) system 9-aGNR. ( 2 ) Structure M-rGOx , undoped 9-aGNR decorated with iron oxide, where one Fe 20 O 32 cluster is employed; the same is used for the adsorption test and collocated at one edge of the graphene nanoribbon. ( 3 ) Structure M-N-rGOx ; a nitrogen-doped 9-aGNR is created by introducing pyridinic defects (N 3 Vc 1 ) along the structure; 14%At of N is reached, which is similar to our experimental N-doped GNS. Then, one Fe 20 O 32 is collocated at one edge of the 9-aGNR. Finally (4) , the structure 2M-N-rGOx , the same N-doped 9-aGNR, structure 3 , is now decorated with two Fe 20 O 32 clusters at each edge of the nanoribbon. We observed that all structures (undoped, N-doped and iron oxide decorated) changes after geometric optimization, resulting in quasi-Archimedean spirals. The final structures are depicted in Supplementary Fig. S15 . We have also defined the rolling energy E roll as E roll = E gnr − E scroll , where E gnr is always the total energy of the flat (step 1) graphene and E scroll is the energy of the rolled structure at one specific rolling step (that is, 2–5), which allows to identify and compare the energy needed to perform the rolling of each structure. The resulting geometries are shown in Supplementary Fig. S15 . Characterization TEM was carried out on a JEOL JEM-1230 transmission electron microscope at 80 keV. HRTEM was carried out on a JEM-2100F at 200 keV with a Gatan Imaging Filter. Scanning transmission electron microscope (STEM) measurements were performed using a Zeiss Merlin FEGSEM (30 kV and a beam current of 210 pA) or a JEM-2100F (200 kV) operated in STEM mode with angular dark-field detector. The Raman spectroscopy was conducted on a Renishaw InVia Raman spectrometer with a charge-coupled device detector (excitation wavelength, 633 nm). The X-ray photoemission spectroscopy was recorded on a Kratos axis ultra delay-line detector electron spectrometer using a monochromatic Al Kα source operated at 150 W. TGA were measured on a Mettler Toledo TGA/DSC 1 LF/948 at a heating rate of 5 °C min −1 for up to 1,000 °C in pure oxygen. X-ray diffraction was carried out on a Siemens D5000 diffractometer with wavelength (Cu Kα) of 1.5418 Å and accelerating voltage 40 kV. A superconducting quantum interference device magnetometer (Quantum Design MPMS 5T) was used for the magnetization measurements. The temperature dependence of the magnetisation was recorded in a field of 1,000 Oe using ZFC and FC protocols ( Fig. 3 ). The ZFC magnetisation was recorded on increasing temperature after cooling the sample in zero field to the lowest temperature of the experiment. The FC magnetisation was recorded on re-cooling the sample in the same magnetic field as in the ZFC measurement. The magnetisation versus field curves ( Supplementary Fig. S10 ) were recorded in the field range 0–1,000 Oe in steps of 100 Oe. How to cite this article: Sharifi, T. et al . Formation of nitrogen-doped graphene nanoscrolls by adsorption of magnetic γ-Fe 2 O 3 nanoparticles. Nat. Commun. 4:2319 doi: 10.1038/ncomms3319 (2013).